Solvent-free aerobic oxidation of hydrocarbons and alcohols with Pd@N-doped carbon from glucose The development of efficient systems for selective aerobic oxidation of hydrocarbons and alcohols to produce more functional compounds (aldehydes, ketones, acids or esters) with atmospheric air or molecular oxygen is a grand challenge for the chemical industry. Here we report the synthesis of palladium nanoparticles supported on novel nanoporous nitrogen-doped carbon, and their impressive performance in the controlled oxidation of hydrocarbons and alcohols with air. In terms of catalytic activity, these catalysts afford much higher turnover frequencies (up to 863 turnovers per hour for hydrocarbon oxidation and up to ~210,000 turnovers per hour for alcohol oxidation) than most reported palladium catalysts under the same reaction conditions. This work provides great potential for the application of ambient air and recyclable palladium catalysts in fine-chemical production with high activity. Historically chemists have realized that one of the cheapest routes to synthesize more useful molecules starting from natural materials was to oxidize those molecules. The selective oxidation of organic compounds, such as alcohols or hydrocarbons, is a primary and essential transformation in organic synthesis and industrial chemistry [1] . Traditionally, various oxidants, such as toxic metal oxides [2] , peroxides (for example, tert-butylhydroperoxide [3] or hydrogen peroxide [4] , [5] ), halides [6] or ozone [7] , etc., were used for these transformations. Compared with those oxidants, undoubtedly, air is the most ubiquitous, atom-economical and environmentally benign oxidant. However, due to the triplet ground state structure of oxygen, air is unreactive and difficult to activate, especially towards the strong C-H bond of hydrocarbons. Nowadays, catalytic oxidations with ambient air as the ultimate oxidant represent one of the most critical technologies in chemical industry. Recently, breakthrough in Pd catalysis provided new opportunities for aerobic oxidation chemistry [8] . From the late 1990s, a number of homogeneous Pd-catalytic systems, such as Pd/coordinating solvent [9] , [10] , Pd/ligand [11] , [12] , [13] , [14] , [15] , have been investigated for aerobic oxidation. Compared with homogeneous catalysts, the heterogeneous catalysts, which are convenient for recycling from the reaction environment and readily used in flow reactors, are more popular, in particular in large-scale production [16] . During the past decade, great progress has also been made in heterogeneous Pd catalysts for oxidation processes, for example, Pd/hydroxyapatite [17] , Pd/mesoporous silicas [18] , [19] polymer-supported Pd [20] , [21] , carbon nanotube-supported Pd [22] , [23] , Pd supported on metal oxide [24] , Pd-containing metal-organic frameworks [25] etc. In the field of oxidation, the current Pd-based catalysis was focusing mainly on the oxidations associating with dehydrogenation processes (alcohol oxidation [26] , [27] , Wacker oxidation [28] , [29] , oxidative couplings [30] , etc.). The aerobic oxidation of hydrocarbons to more functional compounds (aldehydes, ketones, acids or esters), one of the most important processes in petrochemical transformation, has been seldom reported by Pd catalysts [31] , [32] . Recently, the strategy of Au-Pd alloys have enabled O 2 to be used as oxidant in the catalytic oxidation of toluene [33] . However, discovery of active heterogeneous Pd catalysts for the selective oxidation of sp 3 C-H bonds by atmosphere air is still of great importance. The recent fast-growing research upon nanoporous carbon materials offered some unique features (high surface area, thermal and chemical stability and hydrophobic surface properties, etc. ), as a new type of solid supports for heterogeneous catalysis [34] , [35] , [36] . Especially, in the past 5 years, nitrogen-doped carbon materials have became a subject of particular interest to researchers due to their remarkable performance in various applications, such as supercapacitors [37] , catalyst supports [38] , and metal-free oxygen reduction reaction [39] , etc. Doping with the electron-rich nitrogen atoms modifies the surface structure of the carbon materials, with enhanced π-binding ability and improved basicity [40] . The chemical environment of the incorporated nitrogen atom is the key to the control of the properties and it could be distinguished as two major groups: chemical nitrogen (for example, amine or nitrosyl group) and structural nitrogen (for example, pyridinic, pyrollic or quarternary-graphitic nitrogen) ( Supplementary Fig. S1 ). Meanwhile, in homogeneous Pd-catalysed oxidation reactions, nitrogen-based ligands are frequently used with significant promotion effect on the redox process ( Supplementary Fig. S2 ) [30] . Here, similar chemical environments of the nitrogen in the homogeneous nitrogen-based ligands and nitrogen-doped carbon materials make us ask if nitrogen-doped carbon materials can function as ‘heterogeneous N-type ligands’ for Pd-catalysed oxidations, affording some other attractive characters (high stability, recyclability, controllable porous network, etc.) to the ‘ligand family’. An initial experiment supported the hypothesis that nitrogen-doped carbon could accelerate the Pd-mediated aerobic oxidation ( Supplementary Table S1 ), encouraging us to prepare nitrogen-doped carbon as catalyst support. From the standpoint of green and sustainable chemistry, the use of inexpensive, abundant and renewable resources to produce N-doped carbon materials would be highly desirable [41] , [42] . Herein, we wish to report our effort in the synthesis of nanoporous N-doped carbon materials from glucose by hydrothermal carbonization (HTC) process and the utilization of as-prepared material as a basic support to construct Pd catalyst. We also illustrated the successful solvent-free oxidation of hydrocarbons by those Pd catalysts with atmosphere air or molecular oxygen, which at the same time gave high activity in the alcohol oxidation ( Fig. 1 ). The Pd catalyst afforded turnover frequencies (TOFs) that are a factor of ~3–24 greater than those of previous active Pd heterogeneous catalysts (Pd@MgO, Pd@TiO 2 , Pd@CeO 2 , Pd@γ-Al 2 O 3 , Pd@C) in the oxidation of ethylbenzene by air. For the benzyl alcohol oxidation, the Pd catalyst displayed very high activity at 120 °C with 0.1 Mpa O 2 (TOF=~150,000 h −1 ), superior to those results previously reported [17] , [23] , [24] , [26] , [27] . The significantly enhanced activity, utilization of sustainable oxidant, mild reaction conditions and good recyclability made these oxidations highly appealing processes that can address key ‘green chemistry’ priorities in industry. 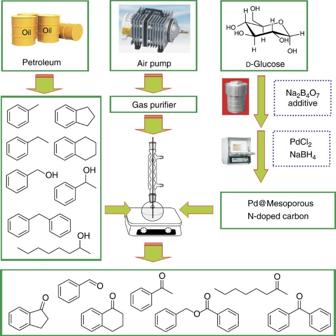Figure 1: Synthetic and catalytic strategy. The substrates and reactors used in the aerobic oxidation, the device for air production and the method for catalyst preparation. Figure 1: Synthetic and catalytic strategy. The substrates and reactors used in the aerobic oxidation, the device for air production and the method for catalyst preparation. Full size image Fabrication of nanostructured nitrogen-doped carbon A modified borax-mediated HTC method was employed in the synthesis of the N-doped carbon materials [43] . As shown in Supplementary Fig. S3 , the N-doped carbon materials were produced in two steps: HTC treatment of D -glucose in the presence of N-containing additives at 200 °C for 8 h; post carbonization of the HTC carbon materials at 550 °C or 1,000 °C under N 2 atmosphere (These carbon materials were denoted as C-Glu A -550, etc., where the subscript word corresponds to the used additive while the last number ‘550’ means the carbonization temperature). The incorporation of ‘N’ into the resulting materials was investigated by elemental analysis ( Supplementary Table S2 ). As expected, the introduction of additive with nitrile group afforded N-doped carbon materials with ~5 wt% nitrogen content. The nature of the nitrogen species on the surface of C-Glu A -550 was further analysed by X-ray photoelectron spectroscopy (XPS) ( Fig. 2a ). The incorporated nitrogen could be regarded as stable structural nitrogen, corresponding to pyridinic nitrogen (39.6%), pyrrolic nitrogen (35.3%) and quaternary-type nitrogen (25.1%). Raman spectroscopy is a powerful tool for identifying carbon materials and detecting the doping effect of heteroatom. The N-doped C-Glu A -550 sample displayed one D band at 1,355 cm −1 and one relatively strong G band at 1,586 cm −1 with I D / I G =0.78 (the intensity ratio of D band to G band), which is higher than that of the C-Glu-550 sample ( I D / I G =0.63), suggesting more structural defects on the N-doped carbon material, possibly induced by the substitutional N species during nitridation ( Supplementary Fig. S4 ) [44] . 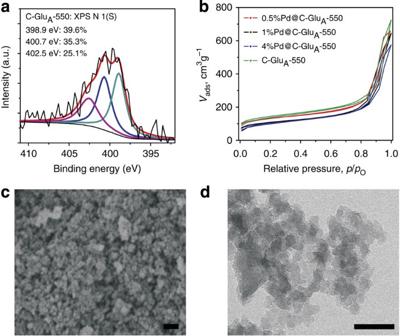Figure 2: Characterizations of representative nitrogen-doped carbon materials. (a) N 1s XPS spectra of N-doped carbon material. (b) Nitrogen adsorption–desorption isotherms for the materials calcined at 550 °C and Pd catalysts. (c) Scanning electron microscopy image from N-doped carbon material. Scale bar, 200 nm. (d) TEM image of the N-doped carbon material. Scale bar, 100 nm. a.u., arbitrary units. Figure 2: Characterizations of representative nitrogen-doped carbon materials. ( a ) N 1s XPS spectra of N-doped carbon material. ( b ) Nitrogen adsorption–desorption isotherms for the materials calcined at 550 °C and Pd catalysts. ( c ) Scanning electron microscopy image from N-doped carbon material. Scale bar, 200 nm. ( d ) TEM image of the N-doped carbon material. Scale bar, 100 nm. a.u., arbitrary units. Full size image Nitrogen adsorption–desorption experiments were performed on all prepared materials and the N-doped carbon, C-Glu A -550, showed a type IV/H 3 adsorption isotherms (BET surface area: 424 m 2 g −1 ) with a sharp condensation of ~0.8 relative pressure, corresponding to the existence of mesopores ( Fig. 2b ; Supplementary Fig. S5 and Table S2 ). X-ray diffraction (XRD) measurements on the prepared samples exhibited a broad reflection around 25° (2 θ ) and a weak reflection around 44° (2 θ ), which could be attributed to the (002) and (100) reflection of the graphitic-type lattice ( Supplementary Fig. S6 ). Moreover, both scanning electron microscopy (SEM) and transmission electron microscopy (TEM) images of the N-doped carbon demonstrated the hierarchical porous network with well-dispersed spherules, which is highly desirable in heterogeneous catalysis ( Fig. 2c , Supplementary Fig. S7 ). It should be noted that this approach could control carbon particle size as small as ~20 nm diameter (calculated from TEM images), much less than conventional HTC carbon materials composed of micrometer-sized spherical particles ( Supplementary Fig. S8 ) [41] , [43] . By combination of excellent porous structure and the nitrogen-doping character, C-Glu A -550 was selected as a support for the preparation of Pd catalysts. Preparation of Pd@nitrogen-doped carbon materials Here, we synthesized systematically Pd@C-Glu A -550 catalysts with different Pd loadings (0.5–4 wt%) by ultrasonic-assisted deposition method [45] . All the frameworks of the Pd catalyst can be assigned to mesoporous materials having type IV adsorption isotherms with a hysteresis loop ( Fig. 2 b). Compared with the support (C-Glu A -550), the as-made Pd@C-Glu A -550 catalysts afforded similar porous nature with reasonable specific surface areas (334–448 m 2 g −1 ) and pore volumes (0.80–0.97 cm 3 g −1 ) ( Supplementary Table S3 ). In the dark-field TEM, the visible particle was identified as Pd nanoparticles by TEM-Energy Dispersive X-ray Detector images ( Supplementary Fig. S9 ). It can be seen that the Pd nanoparticles with a mean size of 5.9 nm were evenly distributed throughout the supporting material ( Fig. 3a , Supplementary Fig. S10 ). The Pd nanoparticles with well-defined lattice fringes in high-resolution TEM (HRTEM) image confirmed the (111) crystal plane of Pd, as the crystal plane spacing was measured as 0.222 nm ( Fig. 3c , Supplementary Fig. S11 ). The Pd 3d XPS spectra in Fig. 3d consists of two asymmetric peaks assigned to Pd 3d 5/2 and Pd 3d 3/2 core levels, which can be fitted using two doublets. The peaks around 336.0 and 341.1 eV are attributed to metallic Pd 0 , while those around 337.6 and 342.4 eV correspond to Pd 2+ species [38] . The Pd dispersion, that is, the fraction of exposed Pd in the 0.5%Pd@C-Glu A -550 catalyst, was determined to be 33.5% by CO adsorption test. Therefore, a high catalytic activity of the Pd@C-Glu A -550 for aerobic oxidation can be expected. 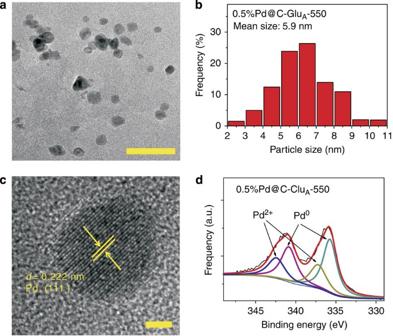Figure 3: Structure characterization of the 0.5%Pd@C-GluA-550 catalyst. (a) TEM image. Scale bar, 20 nm. (b) Pd particle size distribution. (c) HRTEM image. Scale bar, 2 nm. (d) XPS spectra. a.u., arbitrary units. Figure 3: Structure characterization of the 0.5%Pd@C-Glu A -550 catalyst. ( a ) TEM image. Scale bar, 20 nm. ( b ) Pd particle size distribution. ( c ) HRTEM image. Scale bar, 2 nm. ( d ) XPS spectra. a.u., arbitrary units. Full size image Oxidation of indane by Pd catalysts with atmospheric air To investigate the performance of the Pd catalysts in the oxidation of hydrocarbons, solvent-free oxidation of indane with air (1 atm), an important step in the construction of biological and medicinal chemicals [46] , was selected as a model reaction ( Table 1 ). No products can be observed in the blank test at 80 °C (Entry 1, Table 1 ). The C-Glu A -550 support alone did not show any catalytic activity (Entry 2, Table 1 ). Catalysed by 4% Pd@C-Glu A -550, the oxidation afforded a 5.7% indane conversion with 1-indanone as the main product (Entry 3, Table 1 ). As a Pd-based heterogeneous catalyst, the 4% Pd@C-Glu A -550 indeed promoted the air oxidation of sp 3 C-H bond. For comparison, 4% Pd@C-Glu-550 (without nitrogen doping) was tested under the same reaction conditions, and the indane conversion decreased by one third to 3.7% (Entry 4, Table 1 ). Table 1 Oxidation of indane catalysed by Pd catalysts with air. * Full size table The reaction was accelerated at higher temperature, for example, when the temperature was increased to 100 °C, the conversion of indane was significantly improved to 18.4% (Entry 5, Table 1 ). More indane (31.2%) can be transformed into products at 120 °C, affording a TOF of 113 h −1 , though the blank oxidation gave 4.6% indane conversion due to noncatalytic oxidation (Entry 6, Table 1 ). The Pd catalysts with different Pd contents were then investigated in the same reaction process (Entries 7, 8, Table 1 ). Compared with 4% Pd@C-Glu A -550, the 0.5% Pd@C-Glu A -550 showed typically fourfold increase in reaction activity with high selectivity for 1-indanone, exhibiting a TOF of 452 h −1 . In the past decades, the discovery of versatile and efficient Pd/ligand systems largely promoted the Pd-induced oxidations [8] , [15] , [30] , [32] . In our subsequent investigations, various N- or O-type ligands were added into the indane oxidations, testing the effect of different organic ligands on Pd nanoparticles. Among the five additives, it seems that the introduction of 8-hydroxyquinoline and acetylacetone did not affect the catalytic activity so much, while other three additives accelerated the Pd-catalytic oxidations to some degree (Entries 9–13, Table 1 ). In particular, the TOF can be enhanced from 452 h −1 to 863 h −1 by adding a small amount of 2-acetylpyridine (20 mg) in the catalytic system (Entry 13, Table 2 ), suggesting that suitable ligands could also accelerate the heterogeneous Pd-catalysed processes. These organic ligands are expected to destabilize the substrate-Pd intermediate and increase the Pd II /Pd 0 reduction potential, thereby largely promoting the redox process [30] , [32] . Table 2 Oxidation of hydrocarbons and alcohols catalysed by Pd catalysts with air. * Full size table The best advantage of the heterogeneous catalysis was the possibility of recovering and reusing the catalyst after the reaction. The capability of recycling the Pd catalysts was investigated over the oxidation of indane at 80 °C. The results of recycling tests demonstrated that there was almost no significant change in the catalytic activity during the four runs ( Supplementary Fig. S12 ). The liquid phase of the reaction mixture was collected by filtration after the reaction and analysed by inductively coupled plasma—mass spectrometry. Only a very low amount of dissolved palladium (Pd: 2.9 p.p.m., 0.7% of the total palladium in the catalyst) was detected in the solution at the end of the reaction. Especially, when the 0.5% Pd@C-Glu A -550 was removed by a hot filtration in 5 h, the liquid phase did not show any further reaction under the same condition in the subsequent 6 h. All these results suggested that the Pd catalyst is indeed working in a heterogeneous manner, which is a prerequisite for practical applications. Furthermore, when the indane oxidation was carried out in Ar atmosphere, no reaction occurred, giving evidence that air is actually functioning as the oxidant in the system (Entry 14, Table 1 ). When hydroquinone (20 mg), a free radical scavenger, was added into the reaction system, the oxidation was quenched, which implied that the oxidation of indane proceeded through a radical chain pathway (Entry 15, Table 1 ). Oxidation of hydrocarbons and alcohols by Pd catalyst To explore the scope of 0.5% Pd@C-Glu A -550, solvent-free oxidation of some other hydrocarbons were studied under the optimized condition. The oxidation of tetralin to the corresponding products (α-tetralol, α-tetralone) is a key step in the commercial production of α-naphthol and the insecticide [46] , [47] . Catalysed by 0.5% Pd@C-Glu A -550, the tetralin oxidation afforded a TOF of 477 h −1 , with α-tetralol and α-tetralone as the main products (Entry 1, Table 2 ). The catalyst also functioned in the oxidation of diphenylmethane with a moderate TOF of 188 h −1 , possibly due to the steric hindrance (Entry 2, Table 2 ). Ethylbenzene can be selectively oxidized to acetophenone in the presence of 0.5% Pd@C-Glu A -550, giving a TOF of 245 h −1 , yet with some mass loss (note that the air bubbling can take some ethylbenzene away at current reaction conditions) (Entry 3, Table 2 ). It should be mentioned that no hydroperoxide was detected in the above oxidations, probably due to its fast decomposition, converting itself to the major products. Based on these encouraging results, the 0.5% Pd@C-Glu A -550 catalyst was consequently extended to the oxidation of representative alcohols by air. In the presence of 0.5% Pd@C-Glu A -550, benzyl alcohol was smoothly oxidized with benzaldehyde and benzyl benzoate as main products, giving a TOF of 14,802 h −1 (Entry 4, Table 2 ). The formation of benzyl benzoate was due to the esterification reaction of the benzoic acid (over oxidation product of benzaldehyde) and benzyl alcohol, in agreement with previous reported results [48] . The Pd-catalysed oxidation of 1-phenylethanol proceeded very selectively to give acetophenone as product (Entry 5, Table 2 ). This novel catalyst is also suitable for the selective oxidation of 2-octanol to 2-octanone (TOF, 86 h −1 ), which is inactive with the Au-Pd/TiO 2 catalyst (Entry 6, Table 2 ) [26] . Therefore, the present catalytic system has been successfully extended to the alcohol oxidations by air with good activity. Investigation of TOF values under O 2 Given these promising results, the catalytic oxidations were then studied with molecular oxygen as oxidant, which is commonly used in the aerobic oxidation. For the oxidation of benzyl alcohol at 120 °C with 0.1 MPa O 2 , we obtained a TOF of ~150,000 h −1 with 0.5% Pd@C-Glu A -550 catalyst, significantly higher than these reported ones with other active catalysts, such as Au-Pd/TiO 2 (TOF=86,500 h −1 ) (ref. 26 ), Au/TiO 2 (TOF=31,900 h −1 ) (ref. 48 ), Au-Pd/SBA-15 (TOF=27,000 h −1 ) (ref. 49 ), Au/CeO 2 (TOF=12,500 h −1 ) (ref. 50 ), Pd/HAP (TOF=9,800 h −1 ) (ref. 17 ) (Entry 1, Table 3 ). Then, we examined the kinetic effect of varying the availability of oxygen in the benzyl alcohol oxidation. The TOF values became roughly constant in the range of 0.1–1 MPa O 2 , revealing that oxygen pressure does not affect the reaction rates, in some degree (Entries 2, 3, Table 3 ). Under the same conditions with previous reports [17] , [26] , [50] , the TOF of 1-phenylethanol oxidation (160 °C, O 2 0.1 Mpa) reached ~210,000 h −1 , which could be comparable with the result (~269,000 h −1 ) using the Au-Pd/TiO 2 catalyst reported by Hutchings et al. [26] (Entry 4, Table 3 ). Table 3 Oxidation of hydrocarbons and alcohols by Pd catalysts with molecular oxygen. Full size table The aerobic oxidation of ethylbenzene was found to be slower than alcohol oxidation with a TOF of 690 h −1 , and higher O 2 pressure did not lead to higher TOF values in this system (Entries 5, 6, Table 3 ). The aerobic oxidation of toluene is a challenging task in the raw material transformation [33] . In the case of toluene, the Pd catalyst can promote the solvent-free oxidation with benzaldehyde and benzyl benzoate as main products (TOF=4.4 h −1 ) (Entry 7, Table 3 ). With a small amount of 2-acetylpyridine as additive, the TOF value could be enhanced to 18 h −1 , resulting in a 2.7% toluene conversion in 7 h, which further gave evidence that these electron-rich ligands with N − , O − , or a mixture of both types of binding sites hold promising applications in the Pd nanoparticles—catalytic oxidation process (Entry 8, Table 3 ). In the view of TOF values, we can conclude that Pd@C-Glu A -550 is an active heterogeneous catalyst for aerobic oxidation. Study of reaction kinetics The evolution of the catalytic performance with reaction time was then investigated over the solvent-free oxidation of benzyl alcohol, 1-phenylethanol, indane and ethylbenzene with O 2 ( Fig. 4 ). To shorten the reaction time, enhanced amount of Pd catalyst was used in the subsequent tests. All the plots in the Fig. 4 could be fitted with first-order reaction kinetics, and the rate constants were shown in Supplementary Fig. S13 . Under O 2 condition, the benzyl alcohol conversion reached >70% in 7 h with benzaldehyde selectivity ~80% ( Fig. 4a ). The reaction process was also monitored by online Infrared Spectrum (IR) and the benzyl alcohol oxidation showed a maximum reaction rate in the first 10 min ( Supplementary Fig. S14 ). The 1-phenylethanol oxidation proceeded faster, which could be completed in 120 min ( Fig. 4b ). Both alcohol oxidations were performed at 80 °C, and Pd@C-Glu A -550 showed relatively high rate constants k of 0.174±0.013 h −1 and 1.087±0.021 h −1 , for benzyl alcohol and 1-phenylethanol oxidation, respectively. The apparent activation energy (Ea) for the oxidation of benzyl alcohol is extremely low (21.2±2.7 kJ mol −1 ), suggesting an easily initiated reaction ( Supplementary Fig. S15 ). It was observed that more than 60% indane could be smoothly transformed into products in 7 h at 100 °C, with a rate constant k of 0.073±0.004 h −1 ( Fig. 4c ). Because of the inert aliphatic C-H bond (87 kcal mol −1 ), the ethylbenzene oxidation proceeded a little slower, yet with ~40% conversion in 7 h with high selectivity for acetophenone ( Fig. 4d ). 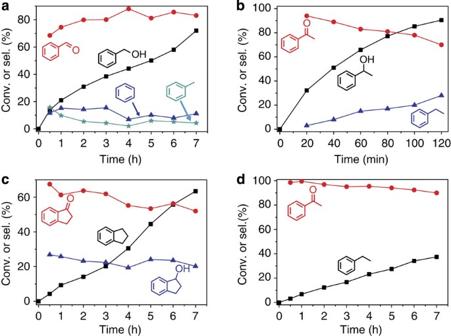Figure 4: Time-activity profile for the aerobic oxidations. The aerobic oxidations of four substrates by Pd@C-GluA-550 catalyst (substrate/metal=~1,000 mol/mol) were recorded. (a) benzyl alcohol 4 ml, 4% Pd@C-GluA-550 0.1 g, 80 °C, O210 ml min−1. (b) 1-Phenylethanol 4 ml, 4% Pd@C-GluA-550 0.1 g, 80 °C, O210 ml min−1. (c) Indane 4 ml, 4% Pd@C-GluA-550 0.1 g, 100 °C, O210 ml min−1. (d) Ethylbenzene 4 ml, 4% Pd@C-GluA-550 0.1 g, 120 °C, O25 ml min−1. Square symbols indicate conversion (conv.), while circle, triangle and pentagon symbols indicate selectivity (sel.). Figure 4: Time-activity profile for the aerobic oxidations. The aerobic oxidations of four substrates by Pd@C-Glu A -550 catalyst (substrate/metal=~1,000 mol/mol) were recorded. ( a ) benzyl alcohol 4 ml, 4% Pd@C-Glu A -550 0.1 g, 80 °C, O 2 10 ml min −1 . ( b ) 1-Phenylethanol 4 ml, 4% Pd@C-Glu A -550 0.1 g, 80 °C, O 2 10 ml min −1 . ( c ) Indane 4 ml, 4% Pd@C-Glu A -550 0.1 g, 100 °C, O 2 10 ml min −1 . ( d ) Ethylbenzene 4 ml, 4% Pd@C-Glu A -550 0.1 g, 120 °C, O 2 5 ml min −1 . Square symbols indicate conversion (conv. ), while circle, triangle and pentagon symbols indicate selectivity (sel.). Full size image Comparing as-made Pd catalyst with other active systems In the next investigation, we tried to carry out the oxidation with some reported active catalysts (Pd@γ-Al 2 O 3 , Pd@MgO, Pd@CeO 2 , Pd@TiO 2 and Pd@C; Supplementary Table S4 ), comparing the catalytic performance of those catalysts with Pd@C-Glu A -550 in atmosphere air. In the ethylbenzene oxidation, these inorganic carriers supported Pd afforded TOFs from 3–21 h −1 under the same reaction conditions (Entries 2–5, Table 4 ). When the commercial Pd@C catalyst was applied in the ethylbenzene oxidation, a moderate TOF (12 h −1 ) was obtained (Entry 6, Table 4 ). It is noteworthy that the TOF value (71 h −1 ) achieved by Pd@C-Glu A -550 are much higher than those tested active catalyst systems (Entry 1, Table 4 ). Further experiments were performed with the oxidation of benzyl alcohol by different Pd catalysts. The Pd@C-Glu A -550 catalyst was shown to outperform other tested Pd catalysts, respecting to their reaction rates ( Supplementary Fig. S16 ). Table 4 Aerobic oxidation of ethylbenzene by various Pd catalysts. * Full size table Based on these catalytic results above, Pd@C-Glu A -550 could be considered as an efficient catalyst in the aerobic oxidation of hydrocarbons and alcohols. From TEM images, it can be observed that, in prepared catalysts, the Pd nanoparticles on nitrogen-doped carbon contained similar sizes with those on nitrogen-free carbon support ( Supplementary Fig. S17 ). Then, we could exclude the effect of the size of Pd nanoparticles on the enhanced catalytic activity, though a recent work revealed that the nitrogen atoms doped in graphene could decrease the size of Au nanoparticles [51] , and the introduction of nitrogen-doped carbon should be the origin of enhancement. The advantages of Pd@C-Glu A -550 are summarized: (1) As indicated by the Raman spectroscopy, the incorporation of nitrogen in the carbon resulted in more structural defects, compared with the nitrogen-free carbon material. Both the incorporated nitrogen atoms and the increased structural defects are expected to anchor substrates efficiently and lead to enhancement of the adsorption of the substrates on the surface of the catalyst, which in principle could boost the oxidation process. Supplementary Fig. S18 depicted the absorption kinetics of benzyl alcohol on the surface of as-synthesized carbon materials. The benzyl alcohol adsorbed at equilibrium over C-Glu A -550 is higher than that on nitrogen-free C-Glu-550. For benzyl alcohol oxidation, the 4% Pd@C-Glu A -550 was found to be indeed more active than 4% Pd@C-Glu-550 ( Supplementary Table S5 ), partly supporting the proposed assumption. In addition, it was reported that the basic support can improve the formation of alcoholate by means of O-H scission in the liquid-phase alcohol oxidation reaction [52] . As a typical basic support, C-Glu A -550 may contribute to O-H scission in the alcohol oxidation, thus promoting the oxidation to some degree. (2) The heterojunction between incorporated nitrogen atoms and Pd species is also an important factor. A careful XPS analysis before and after Pd deposition suggested the surface C/N distribution changed. It was found that the surface nitrogen decreased from 4.9 to 2.2%, implying that the nitrogen sites bound to Pd nanoparticles. The doped nitrogen atoms, especially those with lone pair, might enhance the electron density of Pd 0 , and then promote the oxidative addition of O-H bond or C-H bond to the Pd 0 species, resulting in an increased reaction rate. In summary, we have demonstrated the new Pd catalysts supported on N-doped carbon worked as a highly efficient catalyst in the solvent-free oxidation of hydrocarbons and alcohols with atmosphere air or molecular oxygen. All the porous N-doped carbon materials with high surface area were sustainably prepared from glucose by HTC process. Under O 2 conditions, the 0.5% Pd@C-Glu A -550 afforded high performance in the oxidation of indane (TOF=863 h −1 ), ethylbenzene (TOF=690 h −1 ) and benzyl alcohol (TOF=~150,000 h −1 ). The high catalytic performance has been attributed to the special structure of the catalytic support (nanoporous nitrogen-containing spherules, ~20 nm in diameter) -metal and support-substrate junctions, which leads not only to an electronic activation of the metal nanoparticles but also to an enhancement of the adsorption of substrates and additional electronic activation of the substrates, finally giving rise to fast and selective oxidation. In the indane and toluene oxidation, the combination of organic ligands and Pd@C-Glu A -550 resulted in an interesting synergistic effect that led to enhanced activity, hinting that the introduction of suitable organic ligands could accelerate the heterogeneous Pd catalytic oxidations. Such a correlation with nitrogen and activity presents a simple strategy to tune the activity of supported metal particles through the introduction of nitrogen-doped carbon materials or organic ligands. The recycling test and reaction mixture analysis revealed that the Pd catalyst worked in a heterogeneous manner with negligible Pd leaching. The new method is active, sustainable and recyclable, and especially it allows the utilization of in situ produced air and tolerates many substrates. All these attractive characters make it an ideal environmentally benign chemical process in terms of potential industrial application for this transformation. Materials and general methods Unless otherwise stated, all solvents and chemicals used were of commercially available analytical grade and used without further treatment. N 2 sorption analysis was performed at 77 K using a QUADROSORB SI, equipped with automated surface area and pore size analyser. Before analysis, samples were degassed at 150 °C for 20 h using a masterprep degassing system. The particle morphology was visualized using a Gemini scanning electron microscope. Transmission electron microscopy (TEM) was carried out with a Carl Zeiss Omega 912X at an acceleration voltage of 120 kV. High-Solution TEM (HRTEM), STEM-HAADF and STEM-EDX were performed on Tecnai G2 F30 S-Twin at an acceleration voltage of 300 kV. X-ray powder diffraction (XRD) patterns were measured on a Bruker D8 diffractometer equipped with scintillation counter. Elemental analysis was obtained on a Vario El elemental analyser. The X-ray photoelectron spectra were obtained with an ESCALAB MARK II spherical analyser using a magnesium anode (Mg 1,253.6 eV) X-ray source. The powdered samples were pressed to pellets and fixed to a stainless steel sample holder without further treatment. The XPS spectrum was shifted according to C1s peak being at 288.2 eV, so as to correct the charging effect. The Pd content was measured by inductively coupled plasma analysis and nitric acid (70 wt%, semiconductor grade) was used to dissolve the sample. The CO absorption test was carried out with Quantachrome ChemBET3000, and the catalyst was pre-treated by H 2 (5% in Ar) at 200 °C for 1 h. The online FT-IR spectra were recorded on a Bruker MATRIX-MF. All gas chromatography (GC) experiments were carried out and recorded by GC–MS (Agilent Technologies, GC 6890N, MS 5970). HTC treatment of D -glucose In general, 9.0 g D -glucose, 1.2 g additive (poly(ionic liquid)s) [53] and 0.75 g Borax were dissolved in 30 ml water at room temperature. The mixtures were loaded into a PTFE-lined autoclave and treated at 200 °C for 8 h. The resulting black solids were filtered and washed several times with ethanol and deionized water. The dark brown materials can be obtained by freeze drying. The two carbon materials were denoted as C-Glu-200 and C-Glu A -200, where the subscript word corresponds to the used additive while the last number ‘200’ means the hydrothermal temperature. It should be noted that borax was an important catalyst for the HTC process. Without borax, the HTC of D -glucose resulted in brown solution and no precipitate can be obtained [43] . Synthesis of porous N-doped carbon materials The HTC carbon materials were post-carbonized at the 550 °C (heating rate: 3 K min −1 , holding time: 4 h) and 1,000 °C (heating rate: 3.3 K min −1 , holding time: 1 h) under an inert N 2 atmosphere. After cooling to the room temperature, black carbon materials can be got. Sample labels of final carbons are similar with the HTC carbons except the heat temperature: C-Glu A -550 was C-Glu A -200 additionally treated at 550 °C for 4 h, etc. Preparation of Pd@N-doped carbon materials PdCl 2 (0.5% wt Pd, 3 mg; 1% wt Pd, 5 mg; 4% wt Pd 20.4 mg) and 300 mg C-Glu A -550 were dissolved in 20 ml deionized water. This mixture was stirred at 60 °C for 10 h and cooled to room temperature. Then, the mixture was ultrasonicated for 10 min and NaBH 4 solution (5 equivalent to Pd used, 0.2 mol l −1 ) was added to the solution drop by drop under ultrasonication (in 30 min). The precipitate was centrifuged and washed with deionized water. The resulting Pd catalyst was dried in oven at 80 °C overnight and named as 0.5% Pd@C-Glu A -550, 1% Pd@C-Glu A -550 and 4% Pd@C-Glu A -550. Typical procedure for catalytic oxidation of indane In a typical oxidation, 4 ml indane (calculated by weight) and catalysts used as described in the manuscript were added into a 10-ml three-neck glass reactor, which was fitted with a magnetic stirrer and an air inlet tube. The reaction was performed at an indicated temperature in an oil bath with magnetic stirring (1,000 r.p.m.). A stream of air produced by air pump and gas purifier was conducted into the reaction mixture and controlled by a flowmeter at a constant flow rate (5 ml min −1 ). After completion of the reaction, the reaction mixture was weight and the liquid phase of the reaction mixture was collected by filtration. Then, the liquid mixture (250 μl) and internal standard (Tetralin, 250 μl) was added to 5 ml acetone for GC–MS analysis. Catalytic oxidation of hydrocarbons and alcohols In a typical oxidation, 4 ml substrate (calculated by weight) and catalysts used as described in the manuscript were added into a 10-ml three-neck glass reactor, which was fitted with a magnetic stirrer and an air inlet tube. The reaction was performed at 120 °C in an oil bath with magnetic stirring (stirring rate: 1,000 r.p.m.). A stream of air produced by air pump and gas purifier, or molecular oxygen was conducted into the reaction mixture and controlled by a flowmeter at a constant flow rate (5 ml min −1 ). After completion of the reaction, the reaction mixture weighted and the liquid phase of the reaction mixture was collected by filtration. Then, the liquid mixture (250 μl) and internal standard (250 μl) was added to 5 mL acetone for GC–MS analysis. Catalytic oxidation of alcohols in large scale In a typical oxidation, 50 ml substrate (calculated by weight) and catalysts used as described in the manuscript were added into a 100-ml three-neck glass reactor, which was fitted with a magnetic stirrer and an air inlet tube. The reaction was performed at 120 °C in an oil bath with magnetic stirring (stirring rate: 1,000 r.p.m.). A stream of air produced by air pump and gas purifier, or molecular oxygen was conducted into the reaction mixture and controlled by a flowmeter at a constant flow rate (20 ml min −1 ). After completion of the reaction, the reaction mixture weighed and the liquid phase of the reaction mixture was collected by filtration. Then, the liquid mixture (250 μl) and internal standard (250 μl) was added to 5 ml acetone for GC–MS analysis. Catalytic oxidation under pressured O 2 Those oxidations under pressured O 2 were carried out in a Teflon-lined stainless steel batch reactor. Typically, substrates (calculated by weight) and catalysts used as described in the manuscript were loaded into the reactor (total volume: 100 ml). The reactor was sealed, purged with O 2 to replace the air for three times, increased the O 2 pressure to 1 MPa, and then the reactor was heated to the desired temperature in 20 min. Then, the reaction was carried out for the desired time with magnetic stirring (stirring rate: 1,500 r.p.m.). After reaction, the reactor was placed in ice water to quench the reaction, and the products were analysed by GC–MS with internal standard. Catalyst recycling test When the first oxidation finished, the reaction mixture was centrifuged at 7,000 r.p.m. for 10 min and then the liquid layer was siphoned out. The black solid was washed with ethanol and then centrifuged twice. The catalyst was dried in a vacuum oven at 70 °C for 24 h. Finally, the recovered Pd catalyst was used in the subsequent reaction. How to cite this article: Zhang, P. et al. Solvent-free aerobic oxidation of hydrocarbons and alcohols with Pd@N-doped carbon from glucose. Nat. Commun. 4:1593 doi: 10.1038/ncomms2586 (2013).